Room-temperature photosynthesis of propane from CO2with Cu single atoms on vacancy-rich TiO2 Photochemical conversion of CO 2 into high-value C 2+ products is difficult to achieve due to the energetic and mechanistic challenges in forming multiple C-C bonds. Herein, an efficient photocatalyst for the conversion of CO 2 into C 3 H 8 is prepared by implanting Cu single atoms on Ti 0.91 O 2 atomically-thin single layers. Cu single atoms promote the formation of neighbouring oxygen vacancies (V O s) in Ti 0.91 O 2 matrix. These oxygen vacancies modulate the electronic coupling interaction between Cu atoms and adjacent Ti atoms to form a unique Cu-Ti-V O unit in Ti 0.91 O 2 matrix. A high electron-based selectivity of 64.8% for C 3 H 8 (product-based selectivity of 32.4%), and 86.2% for total C 2+ hydrocarbons (product-based selectivity of 50.2%) are achieved. Theoretical calculations suggest that Cu-Ti-V O unit may stabilize the key *CHOCO and *CH 2 OCOCO intermediates and reduce their energy levels, tuning both C 1 -C 1 and C 1 -C 2 couplings into thermodynamically-favourable exothermal processes. Tandem catalysis mechanism and potential reaction pathway are tentatively proposed for C 3 H 8 formation, involving an overall ( 20 e − – 20 H + ) reduction and coupling of three CO 2 molecules at room temperature. Using sunlight to generate fuels from CO 2 and water has the potential to reduce CO 2 emissions and facilitate the large-scale storage of renewable energy [1] , [2] , [3] , [4] , [5] . Currently, light-driven reduction of CO 2 is mainly limited to two-electron-reduced CO and further reduced C 1 hydrocarbons such as methane (CH 4 ) [6] , [7] and C 2 products such as ethene (C 2 H 4 ) [8] and ethane (C 2 H 6 ) [9] in few cases. However, the formation of C 3 products by artificial photosynthesis is rare [10] , [11] and generally relies on a higher-order reaction pathway that requires the sequential formation of multiple C-C bonds [12] , which involves the integration of two consecutive steps of CO 2 -to-CO and CO-to-C 2+ at different catalytic centres [13] , [14] , [15] , [16] . These C-C couplings are usually challenging endothermic processes with huge uphill energy barriers owing to the high energy levels of the key *C 2 and *C 3 intermediates [17] , [18] , [19] , [20] . These energy barriers result from the lack of effective catalytic centres that can stabilize these multicarbon intermediates [21] , [22] . Single-atom (SA) catalysts with maximum atom utilization efficiency and unique catalytic performance have emerged as an attractive frontier in heterogeneous catalysis [23] , [24] . Atomically thin two-dimensional (2D) materials are suitable platforms to anchor metal SAs [25] , [26] . These 2D single-layer (SL) materials can not only improve the activity of catalytic reactions [27] , but also provide ideal models to gain atomic-level insights into real active sites and reaction mechanisms of catalytic processes through experimental and theoretical techniques [25] , [28] . Herein, we report that implanting Cu SAs in Ti 0.91 O 2 atomic SLs allows the construction of a unique Cu-Ti-V O /Ti 0.91 O 2 -SL photocatalyst for highly efficient and selective conversion of CO 2 into C 3 H 8 . The Cu SA promotes the neighboring Ti 0.91 O 2 to generate oxygen vacancies (V O s) and form a Cu-Ti-V O unit in the Ti 0.91 O 2 matrix. The Cu-Ti-V O /Ti 0.91 O 2 -SL photocatalysis system efficiently converts CO 2 into C 2+ products at room temperature with high electron-based selectivity of 64.8% for C 3 H 8 (product-based selectivity of 32.4%) and 86.2% for overall C 2+ hydrocarbons (product-based selectivity of 50.2%). As suggested by theoretical calculations, the Cu-Ti-V O units may stabilize the key *CHOCO and *CH 2 OCOCO intermediates and reduce their energy levels, tuning both C 1 -C 1 and C 1 -C 2 couplings into thermodynamically favorable exothermal processes. Based on the simulation results, tandem catalytic mechanism and reaction pathway for the production of C 2+ hydrocarbons are proposed, involving an overall 20 e — 20 H + reduction and two sequential C-C coupling processes of three CO 2 molecules ( 3 CO 2 + 20 e − + 20 H + → C 3 H 8 + 6 H 2 O). Our work provides an alternative paradigm for the photoconversion of CO 2 into multicarbon solar fuels, and represents a progressive step toward imitating natural photosynthesis. Formation and characterization of Cu-Ti-V O units Atomically thin layers of Ti 0.91 O 2 -SL were synthesized by exfoliating the layered protonic lepidocrocite-type titanate of H 0.7 Ti 1.825 O 4 [29] , [30] . The absence of peaks in the corresponding X-ray diffraction (XRD) pattern suggests the complete exfoliation into single layers [31] (Supplementary Fig. 1 ). Cu SAs were then implanted in Ti 0.91 O 2 -SL to form Cu-Ti-V O /Ti 0.91 O 2 -SL through a modified wet-chemical route, followed by a rapid thermal treatment (RTT) in an Ar atmosphere [32] (see Methods for details). The amount of Cu loading was detected to be 0.29 wt% by inductively coupled plasma–optical emission spectrometry (ICP-OES). The XRD pattern of Cu-Ti-V O /Ti 0.91 O 2 -SL was similar to that of pristine Ti 0.91 O 2 -SL (Supplementary Fig. 1 ). The thickness of Cu-Ti-V O /Ti 0.91 O 2 -SL was found to be 0.85 nm using atomic force microscopy (AFM) (Supplementary Fig. 2 ), which corresponded closely to the theoretical monolayer thickness (0.75 nm) [30] , [33] , [34] . Field emission-scanning electron microscopy (FE-SEM) and transmission electron microscopy (TEM) images show the ultrathin sheet-like morphology of Cu-Ti-V O /Ti 0.91 O 2 -SL without discernible nanoparticles (NPs) (Fig. 1a–c ), potentially implying the atomic-scale size of the Cu embedded in the Ti 0.91 O 2 matrix. The isolated bright dots in atomic resolution aberration-corrected high angle annular dark-field-scanning transmission electron microscopy (AC HADDF-STEM) images (Fig. 1e ) directly confirm the atomic dispersion of the Cu in the matrix. Energy dispersive X-ray spectroscopy (EDS) mapping (Fig. 1f–i ) indicates that Cu is evenly distributed throughout the atomically thin Ti 0.91 O 2 matrix. Fig. 1: Morphological and structural characterization of Cu-Ti-V O /Ti 0.91 O 2 -SL. a FE-SEM and b , c TEM images, d , e AC HAADF-STEM images, and f – i EDS mapping. Full size image Fourier transforms of the Cu K-edge extended X-ray absorption fine structure (EXAFS) spectra of Cu-Ti-V O /Ti 0.91 O 2 -SL (Fig. 2a ) contain a prominent peak at ~1.56 Å, assigned to Cu-O coordination in the first shell with a coordination number of 4 according to the EXAFS fitting analysis (Supplementary Fig. 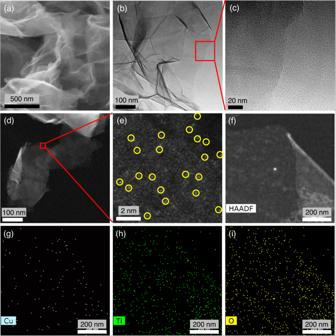Fig. 1: Morphological and structural characterization of Cu-Ti-VO/Ti0.91O2-SL. aFE-SEM andb,cTEM images,d,eAC HAADF-STEM images, andf–iEDS mapping. 3 and Supplementary Table 1 ). The characteristic metallic Cu-Cu bonding at ~2.24 Å is not observed, further validating the single-atom distribution of Cu. A minor scattering peak at ~2.42 Å is attributed to Cu-Ti coordination in the second shell based on the EXAFS fitting results [34] , [35] . The presence of Cu-Ti coordination, originating from the strong electronic interaction between Cu and adjacent Ti atoms, suggests that Cu is present in the atomically dispersed Cu-Ti dual-metal coordination form [36] . Fig. 2: Electronic structure of Cu-Ti-V O /Ti 0.91 O 2 -SL. a Fourier transforms of EXAFS spectra at the Cu K-edge. b EPR spectra. Normalized XANES spectra at the c Cu K-edge and d Ti K-edge. e , f The atomic structure configuration (colour codes: light blue (Ti), blue (Cu), and red (O)). g PDOS and d-band centres of Cu 3 d and Ti 3 d orbitals. h , i COHP between Cu and adjacent Ti. j , k Charge density differences (yellow represents electron accumulation, and purple denotes electron depletion). Full size image The normalized Cu K-edge X-ray absorption near-edge structure (XANES) spectra show that the near-edge absorption energy of Cu-Ti-V O /Ti 0.91 O 2 -SL is higher than that of Cu foil and lies between the energies of Cu 2 O and CuO (Fig. 2c ), indicating that the average oxidation state of Cu is between +1 and +2, which is verified by Cu LMM Auger electron spectra (AES) and Cu 2 p X-ray photoelectron spectra (XPS) as well as the theoretical results (Supplementary Fig. 4a, c ). The near-edge absorption energy and white-line intensity of Ti K-edge XANES for Cu-Ti-V O /Ti 0.91 O 2 -SL are higher than those for Ti 0.91 O 2 -SL (Fig. 2d ), suggesting the presence of Ti species with lower electronic density, which is confirmed by the Ti δ+ (δ > 4) species in Ti 2 p XPS spectra [37] , [38] (Supplementary Fig. 4b ). The formation of these electron-poor Ti centres and the partially oxidized Cu centres proves the electron donation to Cu SAs from the coordinated Ti atoms as a result of the strong electronic interaction in the Cu-Ti dual-metal coordination. 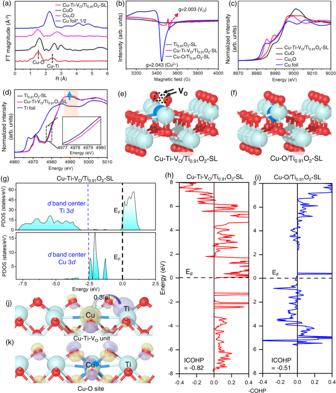Fig. 2: Electronic structure of Cu-Ti-VO/Ti0.91O2-SL. aFourier transforms of EXAFS spectra at the Cu K-edge.bEPR spectra. Normalized XANES spectra at thecCu K-edge anddTi K-edge.e,fThe atomic structure configuration (colour codes: light blue (Ti), blue (Cu), and red (O)).gPDOS and d-band centres of Cu 3dand Ti 3dorbitals.h,iCOHP between Cu and adjacent Ti.j,kCharge density differences (yellow represents electron accumulation, and purple denotes electron depletion). The O 1 s XPS spectrum of Cu-Ti-V O /Ti 0.91 O 2 -SL displays a peak attributed to V O at 531.6 eV [39] , [40] (Supplementary Fig. 5 ). The electron paramagnetic resonance (EPR) spectra also show a V O signal at a g value of 2.003 [40] (Fig. 2b ), suggesting the formation of V O s in Cu-Ti-V O /Ti 0.91 O 2 -SL. In contrast, no V O signal is observed for Ti 0.91 O 2 -SL (Fig. 2b and Supplementary Fig. 5 ). Density functional theory (DFT) computations reveal that the formation energy of V O is 5.66 eV in Ti 0.91 O 2 -SL, while the value sharply decreases to 2.39 eV with Cu anchoring, implying that the introduction of Cu SAs can facilitate the formation of neighboring V O s in the Ti 0.92 O 2 matrix. The strong coordination interaction of the anchored Cu SA with neighboring Ti atoms originates from the presence of V O s. A control sample without V O s (denoted as Cu-O/Ti 0.91 O 2 -SL) was synthesized through a similar RTT in an air atmosphere (see Methods, Fig. 2b, f and Supplementary Fig. 6 for details). The projected density of states (PDOS) of Cu-Ti-V O /Ti 0.91 O 2 -SL (Fig. 2g ) demonstrates that the d -band centre (ɛ d ) of Cu (−2.52 eV) is in good agreement with adjacent Ti (−2.58 eV), inducing a strong electronic coupling effect in the dual-metal sites [36] . The crystal orbital Hamilton population (COHP) between Cu SAs and the closest Ti atoms was then calculated to quantitatively study the intensity of Cu-Ti interactions with and without V O s. The less antibonding orbital populations and a more negative value of integrated-crystal orbital Hamilton population (ICOHP) for Cu-Ti-V O /Ti 0.91 O 2 -SL than Cu-O/Ti 0.91 O 2 -SL prove that the Cu-Ti electronic interaction is much stronger when V O s are present (Fig. 2h, i ). Charge density differences and Bader charge analysis (Fig. 2j ) suggest that 0.3 e − directly transfers to Cu SAs from the neighboring Ti atoms in Cu-Ti-V O /Ti 0.91 O 2 -SL, which causes notable electron accumulation at Cu sites and substantial electron depletion at Ti sites, revealing the asymmetric electron distribution at Cu-Ti coordination. In comparison, without V O s, Cu-O/Ti 0.91 O 2 -SL displays no discernible electron perturbation at Ti sites, and electrons are localized within Cu-O coordination (Fig. 2k ), demonstrating that Cu SAs share negligible interactions with Ti atoms and are in a relatively isolated single-metal form, confirmed by XPS and EPR (Fig. 2b and Supplementary Fig. 6 ). Therefore, both experimental and theoretical analyses indicate that Cu-Ti-V O units are formed in the Ti 0.91 O 2 matrix for Cu-Ti-V O /Ti 0.91 O 2 -SL. In contrast, isolated Cu-O sites are formed in the Ti 0.91 O 2 matrix without V O s for Cu-O/Ti 0.91 O 2 -SL. Photocatalytic CO 2 reduction performance All of the photocatalytic CO 2 reduction metrics reported in this study were measured in CO 2 -saturated acetonitrile aqueous solution (acetonitrile: water = 5:1 by volume) unless otherwise specified, and the testing details are described in the Methods section (Supplementary Fig. 7 ). Unexfoliated layered titanate (denoted as Ti 0.91 O 2 -B) mainly produces CO, with a formation rate of 7.0 μmol g −1 h −1 (Fig. 3b ). Ti 0.91 O 2 -SL displays an enhanced CO production rate of 67.0 μmol g −1 h −1 , indicating that the atomically thin 2D geometry is favorable for the improvement of CO 2 activity through the potential exposure of many rich active sites and a shortened charge-transfer distance from the interior to the surface [26] , [41] . Both CO and CH 4 were detected on Cu-O/Ti 0.91 O 2 -SL with yields of 61.0 and 11.3 μmol g −1 h −1 , respectively. Cu-Ti-V O /Ti 0.91 O 2 -SL exhibit significant yields of C 2 H 4 (7.6 μmol g −1 h −1 ) and C 3 H 8 (13.8 μmol g −1 h −1 ), together with a small amount of CH 4 and trace C 2 H 6 /C 3 H 6 , in addition to CO (18.6 μmolg −1 h −1 ) (Fig. 3a, b ), showing a strong capability of C-C coupling. No H 2 production was detected (Supplementary Fig. 8 ), and O 2 was generated roughly stoichiometrically (Supplementary Fig. 9 ). The quantum efficiency (QE) was obtained 0.48%, 0.15%, and 0.06% at the wavelength of 385, 415, and 520 nm, respectively. A high electron-based selectivity of C 3 H 8 of 64.8% was achieved (32.4% of the product-based selectivity), and that of total C 2+ products was as high as 86.2% (50.2% of the product-based selectivity) (Fig. 3c and Table 1 ). The photocatalytic performance of Cu-Ti-V O /Ti 0.91 O 2 -SL was also tested in pure water. The production rates of all carbon-based products decreased in pure water as compared with those (Supplementary Fig. 10 ). Moreover, the overall selectivity of C 2+ products becomes lower in pure water, and the selectivity of C 3 H 8 is less than C 2 H 4 (Supplementary Fig. 11 ). H 2 is detected with a formation rate of ~2.2 μmol g −1 h −1 in pure water. The improved activity and selectivity are most likely due to the high CO 2 solubility in acetonitrile, which largely increases the local accessibility of CO 2 , thus enhancing the contact between the catalyst and CO 2 molecules to facilitate C-C coupling. 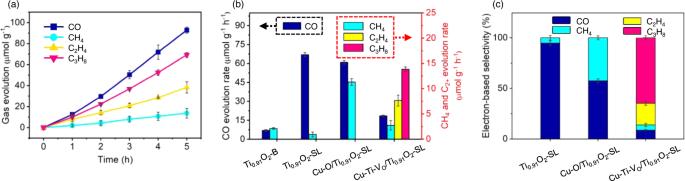Fig. 3: Photocatalytic CO2reduction performance in acetonitrile aqueous solution. aPhotocatalytic product evolution as a function of light irradiation times on Cu-Ti-VO/Ti0.91O2-SL.bProduct formation rates andcelectron-based selectivity on Ti0.91O2-SL, Cu-O/Ti0.91O2-SL, and Cu-Ti-VO/Ti0.91O2-SL. (Error bars indicate standard deviations.). To the best of our knowledge, the efficiency and selectivity of C 3 H 8 production in our work outperform most of the reported photocatalysts in acetonitrile medium, and also rank among the top of the reported C 2+ production photocatalysts in non-acetonitrile medium (Supplementary Table 3 ). Fig. 3: Photocatalytic CO 2 reduction performance in acetonitrile aqueous solution. a Photocatalytic product evolution as a function of light irradiation times on Cu-Ti-V O /Ti 0.91 O 2 -SL. b Product formation rates and c electron-based selectivity on Ti 0.91 O 2 -SL, Cu-O/Ti 0.91 O 2 -SL, and Cu-Ti-V O /Ti 0.91 O 2 -SL. (Error bars indicate standard deviations.). Full size image Table 1 Selectivity of different products on Ti 0.91 O 2 -SL, Cu-O/Ti 0.91 O 2 -SL, and Cu-Ti-V O /Ti 0.91 O 2 -SL. a Full size table The substantially suppressed CO production and increased C 2+ production on Cu-Ti-V O /Ti 0.91 O 2 -SL, compared with pristine Ti 0.91 O 2 -SL, imply that the formation of C 2+ products is potentially derived from the coupling depletion of the *CO intermediate. CO was used to substitute CO 2 as the starting reactant on Cu-Ti-V O /Ti 0.91 O 2 -SL, and a considerable amount of C 3 H 8 and C 2 H 4 was indeed detected (Supplementary Fig. 12 ), further confirming *CO as an important intermediate for the present C 2+ products. The distinctive CO 2 photoreduction activity and high selectivity of C 3 H 8 and total C 2+ products are still well maintained after three-cycle tests of 15 h in total (Supplementary Figs. 13 and 14 ), and the post-reaction characterizations of Cu-Ti-V O /Ti 0.91 O 2 -SL display no obvious structural and morphological changes (Supplementary Figs. 15 – 17 ), demonstrating the excellent stability of the catalyst. Notably, with the decrease in the Cu loading amount, the C 2+ yield declines as the lower Cu loading reasonably reduces the number of Cu-Ti-V O units, restraining C-C coupling (Supplementary Figs. 18 and 19 ). Moreover, higher Cu loading results in Cu aggregation into nanoclusters (NCs) and nanoparticles (NPs), subsequently lowering the selectivity of C 2+ products, which is probably due to the weaker coupling interaction between Cu and the Ti 0.91 O 2 matrix as the metal particle size increases [42] , [43] (Supplementary Fig. 18 ). A series of control experiments were performed in the absence of illumination, the catalyst or CO 2 , and no detectable CO or other hydrocarbon products were detected. The 13 CO 2 isotope labeling experiment and the time profile of relative abundance of 13 C labeled products confirm that the carbon source for CO and other hydrocarbon products originates from the input CO 2 gas [44] (Supplementary Figs. 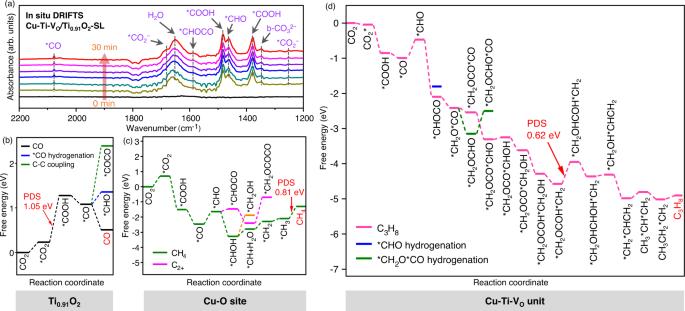Fig. 4: Mechanism studies of CO2reduction on Cu-Ti-VO/Ti0.91O2-SL. aIn situ DRIFTS spectra of the photocatalytic CO2reduction on Cu-Ti-VO/Ti0.91O2-SL. Gibbs free energy diagrams of CO2reduction onbTi0.91O2matrix,cCu-O site, anddCu-Ti-VOunit. 20 and 21 , and Supplementary Table 4 ). The light utilization and the charge carrier dynamics of the as-prepared catalysts were studied. The absorption edge of single-layer Ti 0.91 O 2 -SL displays a blue shift compared with layered Ti 0.91 O 2 -B due to the quantum confinement effect of monolayer structure, while the light absorption is enhanced after implantation of Cu single atoms (Supplementary Fig. 22 ). Photoelectrochemical (PEC) measurements confirm the enhanced charge separation and migration efficiency of Cu-Ti-V O /Ti 0.91 O 2 -SL, ascribed to the 2D atomically-thin structure, which effectively shortens the charge transfer distance from body to surface and lowers charge recombination possibility (Supplementary Fig. 23 ). The fast charge carrier dynamics of Cu-Ti-V O /Ti 0.91 O 2 -SL is kinetically favorable for the multi-electron reactions of generating C 2+ products. Moreover, CO 2 adsorption isotherms reveal that Cu-Ti-V O /Ti 0.91 O 2 -SL possesses the highest CO 2 uptake capacity, which is a priority for CO 2 activation and reduction (Supplementary Fig. 24 ). Theoretical calculations for CO 2 photoreduction mechanism The substantial suppression of CO production and promotion of C 2+ production by Cu-Ti-V O /Ti 0.91 O 2 -SL, in sharp contrast to pristine Ti 0.91 O 2 -SL, has demonstrated the key role of Cu-Ti-V O units in coupling *CO intermediates into C 2+ products. In fact, our in situ diffuse reflectance Fourier transform infrared spectroscopy (DRIFTS) characterization using 12 CO 2 and 13 CO 2 has detected the formation of the key *COOH, *CO, *CHO, and *CHOCO intermediates on Cu-Ti-V O /Ti 0.91 O 2 -SL (Fig. 4a , Supplementary Figs. 25 and 26 , and Supplementary Note 1 ), indicating the coupling of *CO into *CHOCO intermediates. However, it is not feasible to experimentally establish a direct spatial correlation between the active sites and the evolution of reaction intermediates to allow for deeper understanding on CO 2 photoreduction mechanism on atomic level. For this reason, density functional theory (DFT) calculations with a computational hydrogen electrode (CHE) model [45] , [46] was employed in an attempt to describe one potential mechanism for the reaction of CO 2 -to-C 2+ products on Cu-Ti-V O /Ti 0.91 O 2 -SL. Fig. 4: Mechanism studies of CO 2 reduction on Cu-Ti-V O /Ti 0.91 O 2 -SL. a In situ DRIFTS spectra of the photocatalytic CO 2 reduction on Cu-Ti-V O /Ti 0.91 O 2 -SL. Gibbs free energy diagrams of CO 2 reduction on b Ti 0.91 O 2 matrix, c Cu-O site, and d Cu-Ti-V O unit. Full size image In the calculations, Cu-Ti-V O /Ti 0.91 O 2 -SL are featured with two types of catalytic centres for CO 2 reduction: the Cu atom-free Ti 0.91 O 2 matrix domain and the Cu-Ti-V O unit domain. On Ti 0.91 O 2 domain, CO 2 is reduced to *CO through *COOH intermediate [47] (Fig. 4b and Supplementary Fig. 27 ). DFT results suggest the easy desorption of *CO on Ti 0.91 O 2 matrix rather than further hydrogenation or C-C coupling (Supplementary Note 2 ), consistent with the experimental observation of the dominant CO product on pristine Ti 0.91 O 2 -SL. On Cu-Ti-V O unit domain, the absorbed CO 2 is firstly converted to *CHO through *COOH and *CO intermediates [48] (Supplementary Fig. 27 ). Then, the *CHO at Cu-Ti-V O unit may couple with the CO diffusing from neighboring Ti 0.91 O 2 domain to generate *CHOCO [49] , [50] , [51] with free energy change of −1.63 eV (see Supplementary Note 3 for more details about potential pathways). The following C 1 -C 2 coupling (*CH 2 OCO + *CO → *CH 2 OCOCO) is also calculated to be a thermodynamically-favorable exergonic reaction (−0.13 eV) (Supplementary Note 3 ). As a contrast, it is worth noting that on the Cu-O site without Vos, C-C coupling processes are found to be challenging owing to the large uphill energy changes, while the hydrogenation of *CO into CH 4 is more preferred (Fig. 4c ) [52] , [53] . Meanwhile, for Cu-Ti-V O unit, some of the *C 2 species will continue to hydrogenate through a series of proton-electron steps to form C 2 H 4 . The free energy change of the potential determining step (PDS) is calculated as 0.62 eV for the C 3 H 8 formation pathway (Fig. 4d ) and 0.90 eV for the C 2 H 4 formation pathway (Supplementary Fig. 28 ), suggesting the easier formation of C 3 H 8 than C 2 H 4 . This is in accordance with our photocatalytic experimental observation of the higher yield of C 3 H 8 than C 2 H 4 on Cu-Ti-V O /Ti 0.91 O 2 -SL. The overall reaction pathway for the reduction of CO 2 to C 3 H 8 and C 2 H 4 over Cu-Ti-V O /Ti 0.91 O 2 -SL is tentatively described in Supplementary Fig. 29 . In summary, the above results suggest a tandem catalysis mechanism [13] , [14] , [15] , [16] , [54] , [55] , [56] , where the Cu-free Ti 0.91 O 2 matrix may be preferential to participate in the reduction of CO 2 to CO, and Cu-Ti-V O unit is more beneficial to the exergonic C-C coupling to C 2+ products (Supplementary Fig. 30 ). The above result suggests favorable exergonic reactions for both C 1 -C 1 and C 1 -C 2 couplings on Cu-Ti-V O unit, which is in sharp contrast with Cu-O sites and other previously-reported catalysts with challenging endergonic C-C couplings [17] , [18] , [19] , [20] . Such downhill energy changes of C-C coupling on Cu-Ti-V O unit are probably owing to the low energy levels of the *CHOCO and *CH 2 OCOCO intermediates (Supplementary Fig. 31 ). A stable multiple-bonding configuration containing one Cu-C bond and two Ti-O bonds is built for the adsorption of *CHOCO on Cu-Ti-V O unit (Supplementary Fig. 32 ). Moreover, a five-membered ring is formed between *CH 2 OCOCO and Cu-Ti-V O unit, largely alleviating the electron accumulation and relaxing the intermolecular and intramolecular electrostatic repulsion (Supplementary Fig. 33 ). The electronic and geometric effect of Cu-Ti-V O unit may jointly stabilize these key *C 2+ intermediates and lower their adsorption energy levels to promote C-C couplings. A unique Cu-Ti-V O unit in atomically thin Ti 0.91 O 2 monolayer nanosheets was developed for highly efficient and selective photoconversion of CO 2 to C 3 H 8 . Theoretical calculations suggested that the Cu-Ti-V O unit, as a favorable reaction centre for both C 1 -C 1 and C 1 -C 2 couplings, can effectively facilitate the multistep photocatalytic reduction of CO 2 by reducing the energy levels of the key *CHOCO and *CH 2 OCOCO intermediates via electronic and geometric effects. A tandem mechanism and possible reaction pathway are proposed for the conversion of CO 2 to C 3 H 8 . The results of our study may open an alternative avenue for designing and synthesizing tandem photocatalysts with dual-metal active sites and coordination vacancies that modulate the behavior of reaction intermediates for the production of multicarbon fuels driven by light. Synthesis of catalysts Cu-Ti-V O /Ti 0.91 O 2 -SL: Single-layer Ti 0.91 O 2 nanosheets were synthesized according to previous literature [29] , and the specific procedure is presented below. The parent Cs compound, Cs 0.7 Ti 1.825 O 4, was obtained by repeating twice the heat treatment (800 °C, 20 h) for the mixture of 10 mmol Cs 2 CO 3 and 53 mmol anatase TiO 2 . The interlayer Cs ions were extracted by stirring 5 g of the as-prepared Cs 0.7 Ti 1.825 O 4 in 500 mL of 1 M HCl solution for 24 h. After four cycles of acid exchange, the solid was washed with DI water to remove excess acid and then dried in a freeze dryer. Layered protonic lepidocrocite-type titanate of H 0.7 Ti 1.825 O 4 was obtained. 0.4 g of the as-prepared layered H 0.7 Ti 1.825 O 4 was shaken with 100 mL of 0.08 M tetrabutylammonium (TBA) hydroxide aqueous solution for a week to produce stable colloidal suspensions of atomically thin Ti 0.91 O 2 single layers. The colloidal suspensions were then dried in a freeze dryer. The Cu-en precursor was prepared by mixing 30 mL of 0.025 g/L CuCl 2 ‧2H 2 O aqueous solution with 360 μL of ethanediamine (en) at room temperature. Then, this Cu-en precursor was added to 7 g of the as-prepared colloidal suspensions of single-layer Ti 0.91 O 2 . After stirring for 5 h, the solid was filtrated, washed with deionized water, and dried in a freeze dryer to obtain a single-layer Cu-en/Ti 0.91 O 2 sample. Then, the Cu-Ti-V O /Ti 0.91 O 2 -SL sample was prepared by rapid thermal treatment (RTT) of single-layer Cu-en/Ti 0.91 O 2 in an Ar atmosphere at 500 °C for 1 min [32] . Briefly, the powders were put into a quartz tube, which was then inserted into a tube furnace preheated to 500 °C. Under Ar flow, the powders were kept at that temperature for 1 min, and then the quartz tube was quickly removed and rapidly cooled to room temperature. Cu-O/Ti 0.91 O 2 -SL: The sample was prepared by the same method as Cu-Ti-V O /Ti 0.91 O 2 -SL, except that the RTT process was conducted in an air atmosphere. Cu-Ti-V O /Ti 0.91 O 2 -SL (lower): The sample was prepared by the same method as Cu-Ti-V O /Ti 0.91 O 2 -SL, except that an aqueous solution of 0.0125 g/L CuCl 2 ‧2H 2 O was used. Cu NC/Ti 0.91 O 2 -SL: The sample was prepared by the same method as Cu-Ti-V O /Ti 0.91 O 2 -SL, except that an aqueous solution of 0.1 g/L CuCl 2 ‧2H 2 O was used. Cu NP/Ti 0.91 O 2 -SL: The sample was prepared by the same method as Cu-Ti-V O /Ti 0.91 O 2 -SL, except that an aqueous solution of 0.2 g/L CuCl 2 ‧2H 2 O aqueous was used, and RTT was maintained at 10 min. Ti 0.91 O 2 -B: The sample was prepared by treating layered protonic lepidocrocite-type titanate of H 0.7 Ti 1.825 O 4 with the same RTT process as used for Cu-Ti-V O /Ti 0.91 O 2 -SL. Characterization XRD data were measured on an X-ray diffractometer (Rigaku Ultima III, Japan) by Cu-Kα radiation (λ = 0.154178 nm) at 40 kV and 40 mA with a scan rate of 5° min −1 . AFM analysis was performed on an MFP3D microscope (Asylum Research, MFP-3D-SA, USA) with a cantilever operating in tapping mode. The morphology was characterized by FE-SEM (FEI NOVA NANOSEM 230). TEM images were taken on an FEI Tecnai F20 TEM apparatus. Atomic-resolution STEM-HAADF images were obtained on a double spherical aberration-corrected STEM/TEM FEI Titan3 Cubed 60–300, and the samples were suspended on micron-scale carbon grids of Mo mesh. The Cu concentration was determined by ICP–OES with an Avio200 instrument. The XAFS spectra (Cu K-edge and Ti K-edge) were collected at the 1W1B station at the Beijing Synchrotron Radiation Facility (BSRF). The storage rings at BSRF were operated at 2.5 GeV with an average current of 250 mA. Using a Si (111) double-crystal monochromator, the data collection was conducted in transmission/fluorescence mode using an ionization chamber. All spectra were collected under ambient conditions. The EXAFS data were processed according to standard procedures using the ATHENA module implemented in the IFEFFIT software package. The k 3 -weighted EXAFS spectra were obtained by subtracting the postedge background from the overall absorption and then normalizing with respect to the edge jump step. Subsequently, k 3 -weighted χ(k) data of the Cu K-edge underwent Fourier transform to real (R) space using Hanning windows (dk = 1.0 Å −1 ) to separate the EXAFS contributions from different coordination shells. To obtain the quantitative structural parameters around the central atoms, least squares curve parameter fitting was performed using the ARTEMIS module of IFEFFIT software packages. The chemical states of the samples were detected by XPS and AES, which were equipped with an ultrahigh vacuum Thermo Fisher Scientific electron spectrometer by using Al Kα radiation (1486.6 eV) as the X-ray source, and the binding energies were calibrated according to the C 1 s peak of adventitious carbon at 284.6 eV. The in situ DRIFTS spectra were obtained on a Bruker IFS 66 v FT spectrometer with Harrick diffuse reflectance with ZnSe and quartz windows at BL01B in NSRL, Hefei. Measurements of photocatalytic CO 2 reduction Photocatalytic CO 2 reduction experiments were performed in a Pyrex reaction vessel with a top irradiation window. Typically, 10 mg of photocatalyst powder was suspended in a 15 mL CO 2 -saturated solution containing 12.5 mL acetonitrile and 2.5 mL H 2 O in a 166 mL quartz reaction cell. Before illumination, the system was filled with CO 2 (purity >99.999%) to 1 atm. The reactor was then irradiated by a 300 W Xe lamp (PerfectLight, PLS-SXE300). During irradiation, 0.1 mL of gas was collected from the reaction headspace every hour, and the gaseous products were analysed by using gas chromatography (GC-2014C, Shimadzu Corp., Japan). The isotope experiment was conducted using 13 CO 2 as feedstock, and the products were analysed using gas chromatography–mass spectrometry (7890 A and 5975 C, Agilent). The quantum efficiency was evaluated using a LED lamp (PerfectLight) with the wavelength of 385,415, or 520 nm as the light source. The electron-based selectivity of C 3 H 8 was calculated using (1): 
    Sel_electron(C_3H_8)=(n (C_3H_8)× 20/n(CO)× 2+n(CH_4)× 8+n(C_2H_4)× 12+n(C_3H_8)× 20)× 100%
 (1) The product-based selectivity of C 3 H 8 was calculated using (2): 
    Sel_product(C_3H_8)=(n(C_3H_8)/n(CO)+n(CH_4)+n(C_2H_4)+n(C_3H_8))× 100%
 (2) The electron-based selectivity of C 2+ products was calculated using (3): 
    Sel_electron(C_2+)=(n(C_2H_4)× 12+n(C_3H_8)× 20/n(CO)× 2+n(CH_4)× 8+n(C_2H_4)× 12+n(C_3H_8)× 20)× 100%
 (3) The product-based selectivity of C 2+ products was calculated using (4): 
    Sel_product(C_2+)=(n(C_2H_4)+n(C_3H_8)/n(CO)+n(CH_4)+n(C_2H_4)+n(C_3H_8))× 100%
 (4) where n is the formation rate. The quantum efficiency was calculated using (5): 
    QE=N(CO)× 2+N(CH_4)× 8+N(C_2H_4)× 12+N(C_3H_8)× 20/N(photon)× 100%
 (5) where N is the number of evolved gas molecules or incident photons. Computational details All calculations were performed based on density functional theory (DFT) through the Vienna ab initio Simulation Package (VASP) [57] . Projector-augmented-wave (PAW) pseudopotentials [58] were used to treat the core electrons, while interactions between electrons were described by the Perdew-Burke-Ernzerhof (PBE) [59] exchange-correlation functional of the generalized gradient approximation (GGA). For all the calculations, the vacuum space in the z-direction was 20 Å to avoid potential interactions between periodic surfaces. The DFT-D3 method of Grimme [60] was applied to describe the van der Waals dispersion forces. DFT + U approach [61] , [62] with U = 3.5 eV was considered to evaluate the influence of strongly correlated d electrons on the calculated free energies. According to our previous report [63] , the results of calculated free energies obtained from DFT + U and DFT are consistent. Therefore, regular DFT was employed in this work. The Monkhorst-Pack k-point grid with 3 × 3 × 1 mesh was applied until the maximal forces on each ion were smaller than 0.02 eV/Å. The convergence criterion of the energy was set to 10 −4 eV, and a cut-off energy of 450 eV was used for the plane wave expansion. The Gibbs free energy change (Δ G ) was defined as follows [45] , [64] : 
    Δ G=Δ E+ΔE_ZPE-TΔ S
 (6) where Δ E is the energy difference between the reactants and product obtained through DFT calculations. Δ E ZPE and Δ S are the changes in the zero-point energies (ZPE) and entropy [65] . T represents the temperature and was set as 298.15. Statistics & reproducibility No statistical method was used to predetermine the sample size. No data were excluded from the analyses. The experiments were not randomized.